The allosteric vestibule of a seven transmembrane helical receptor controls G-protein coupling Seven transmembrane helical receptors (7TMRs) modulate cell function via different types of G proteins, often in a ligand-specific manner. Class A 7TMRs harbour allosteric vestibules in the entrance of their ligand-binding cavities, which are in the focus of current drug discovery. However, their biological function remains enigmatic. Here we present a new strategy for probing and manipulating conformational transitions in the allosteric vestibule of label-free 7TMRs using the M 2 acetylcholine receptor as a paradigm. We designed dualsteric agonists as 'tailor-made' chemical probes to trigger graded receptor activation from the acetylcholine-binding site while simultaneously restricting spatial flexibility of the receptor's allosteric vestibule. Our findings reveal for the first time that a 7TMR's allosteric vestibule controls the extent of receptor movement to govern a hierarchical order of G-protein coupling. This is a new concept assigning a biological role to the allosteric vestibule for controlling fidelity of 7TMR signalling. Seven transmembrane helical receptors (7TMRs; G-protein-coupled receptors) are embedded into the membrane of almost all cells and are essential for orchestrating the function of cells in order to maintain homoeostasis of the organism and its adaptation to environmental changes. In addition, modulation of 7TMR function by drugs is a mainstay for the prevention and treatment of disease [1] . The human genome encodes about 800 7TMRs with the rhodopsin-like class A receptors representing the quantitatively dominating subfamily, which include aminergic and cholinergic receptors [2] . 7TMR activation by an extracellular stimulus is communicated to the cell by a conformational rearrangement of the intracellular domain region that mediates recruitment and activation of adaptor proteins. These proteins control the activity of intracellular signalling pathways and include guanylnucleotide-binding proteins (G proteins) and β-arrestins [3] . Heterotrimeric G proteins are subdivided into four families based on sequence homologies and functional similarities of their Gα subunits, G i/o , G s , G q/11 and G 12/13 (ref. 4 ). These can be addressed selectively, but often an endogenous activator-bound 7TMR has efficacy to activate more than one class of G protein, which is referred to as promiscuous signalling. Remarkably, especially from a therapeutic point of view, chemically modified artificial ligands may engender more precise signalling than the endogenous activator molecule, which is designated as biased signalling, functional selectivity or signal trafficking [5] , [6] , [7] . It is likely that the signalling repertoire of a 7TMR corresponds to ensembles of possible conformations of the receptor protein, and that a biased activator allows only for a subset of possible receptor conformations [8] . Crystal structures of 7TMRs give fascinating insight into the conformational rearrangements that accompany inactive-to-active transitions [9] , [10] , [11] . However, the molecular principles by which a receptor protein translates the chemical properties of a ligand into a signalling fingerprint are still unresolved [12] . Accumulating evidence suggests that there is no consensus sequence for adaptor protein-coupling specificity on the level of the intracellular domains [13] , and, in line with this notion, signalling is often promiscuous. On the level of the helical bundle region, 7TMR structure is highly conserved, which would correspond well to a general activation mechanism [14] but not to coupling selectivity. In the extracellular loop region, however, there is rather high variability between primary structures. Remarkably, a ligand-dependent conformational coupling from the orthosteric site to the extracellular loop region has recently been described [15] . Intriguingly, class A 7TMRs harbour allosteric vestibules in the extracellular entrance of their ligand-binding cavities, which receive high attention as new targets for drug discovery [16] . However, until now, their biological function is poorly understood. The question therefore arises whether the extracellular domains hold a function in controlling intracellular signalling of a 7TMR. We took advantage of a new strategy for probing the allosteric vestibule's role for signal trafficking using the M 2 acetylcholine (ACh) receptor as a paradigm for small ligand 7TMRs. Muscarinic ACh receptors are important targets for novel drugs with improved selecitivtiy [17] , and in particular, fundamental insights of 7TMR function have first been achieved with this receptor. These include the discovery of 7TMR allosterism [18] , the establishment of the ternary complex model of allosteric interactions [19] , its proof with a radiolabelled allosteric probe [20] and the identification of allosteric key epitopes as well as their spatial orientation within the allosteric vestibule [21] , [22] , [23] . We designed a set of 'tailor-made' chemical probes, referred to as dualsteric agonists [24] , to trigger graded receptor activation from the ACh-binding site (that is, the orthosteric site) while simultaneously restricting spatial flexibility of the receptor's extracellular allosteric vestibule. Evaluation of probe actions in this study in a broad array of signalling readouts, including those in a space-providing 'rescue mutant', show that the allosteric vestibule of the M 2 receptor controls the extent of receptor movement thereby governing a hierarchical order of intracellular adaptor protein recruitment. This is a new concept assigning an unprecedented biological role to the allosteric vestibule for controlling fidelity of receptor signalling of a small molecule 7TMR. Strategy for new chemical tool design Muscarinic ACh receptors belong to the class A of G-protein-coupled receptors, which bind their endogenous agonist deep in the ligand-binding cleft lined by transmembrane helical domains [25] , [26] , [27] . Asp103 3.32 ( Fig. 1a ) serves as a docking point for the positively charged nitrogen of ACh. Iperoxo (( 1 ) in Fig. 1b ), the orthosteric building block of the dualsteric compounds, is a super-potent muscarinic agonist characterized by an affinity-enhancing Δ 2 -isoxazoline ring system and was re-synthesized as previously described [28] . Iperoxo is 100-fold more potent than ACh as reported below and was chosen as the orthosteric building block of the dualsteric probes to ensure high-fidelity receptor activation via the orthosteric-binding site. To study the role of the allosteric substituent for signalling (shaded grey in Fig. 1b ), iper-6 (( 2 ) in Fig. 1b ) was synthesized ( Supplementary Methods ), which carries the linker chain without the spacious allosteric building blocks. The allosteric phthalimide building block contained in iper-6-phth (( 3 ) in Fig. 1b ) has no efficacy for receptor activation [29] and binds to M 2 -W422 7.35 at the beginning of TM7 and to M 2 -Y177 5.32 in the extracellular loop 2 ( Fig. 1a ) [21] , [22] , [23] . These two amino acids are located opposite to each other in the depth of the allosteric vestibule in close vicinity to the subjacent orthosteric site [23] . The crystal structure of the inactive antagonist-bound M 2 receptor proves the location of M 2 -Y177 5.32 and M 2 -W422 7.35 outside of and above the aromatic cage that encloses the orthosteric ligand, respectively [25] . Docking simulations show that the allosteric building block protrudes to the level of M 2 -W422 7.35 (ref. 24 ). If this binding topography causes a signalling bias, enlargement of the substituent to naphthalimide (in iper-6-naph, ( 5 ) in Fig. 1b ), which by itself also has no efficacy for receptor activation [29] , should further impair signalling. Iper-6-phth and iper-6-naph were re-synthesized precisely as described previously [24] . In contrast, elongation of the hexamethylene middle chain to octamethylene, as realized in the newly synthesized iper-8-phth and iper-8-naph (( 4 ) and ( 6 ) in Fig. 1b , respectively, Supplementary Methods ), would be expected to restore the signalling by shifting the spacious substituent outward of this critical region. 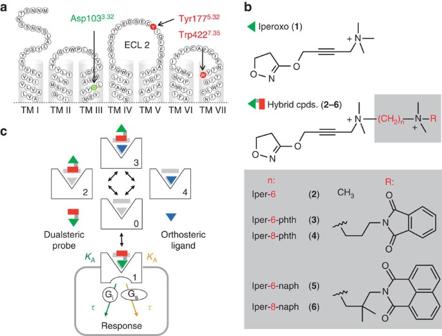Figure 1: Receptor binding poses of dualsteric probes. (a) Snake-like plot of the outer loop region of the muscarinic M2receptor along with the flanking alpha-helical domains. Arrows indicate essential epitopes for orthosteric (green) and allosteric (red) ligand binding. (b) Dualsteric hybrid design: the super high-affinity orthosteric muscarinic agonist iperoxo is linked via a hexamethylene- or octamethylene-spacer with allosteric inverse agonistic phthalimide or naphthalimide moieties. (c) Receptor binding poses of dualsteric probes in the absence (1,2) and presence (3) of an orthosteric ligand. With the hybrid design of this study, only the dualsteric binding mode (1) leads to receptor activation and downstream signalling. The coupling efficiencyτquantifies the efficacy with which agonist-occupied receptors activate Giand Gssignalling. The coupling of either Gior Gsproteins to the M2receptor affects the binding constantKAof the dualsteric agonist. Figure 1: Receptor binding poses of dualsteric probes. ( a ) Snake-like plot of the outer loop region of the muscarinic M 2 receptor along with the flanking alpha-helical domains. Arrows indicate essential epitopes for orthosteric (green) and allosteric (red) ligand binding. ( b ) Dualsteric hybrid design: the super high-affinity orthosteric muscarinic agonist iperoxo is linked via a hexamethylene- or octamethylene-spacer with allosteric inverse agonistic phthalimide or naphthalimide moieties. ( c ) Receptor binding poses of dualsteric probes in the absence (1,2) and presence (3) of an orthosteric ligand. With the hybrid design of this study, only the dualsteric binding mode (1) leads to receptor activation and downstream signalling. The coupling efficiency τ quantifies the efficacy with which agonist-occupied receptors activate G i and G s signalling. The coupling of either G i or G s proteins to the M 2 receptor affects the binding constant K A of the dualsteric agonist. Full size image Probe binding to cell surface hM 2 -receptors Ligand–receptor interactions in live CHO cells transfected to stably express hM 2 receptors (CHO-hM 2 cells) were measured using the non-permeant orthosteric radioligand [ 3 H]- N -methylscopolamine ([ 3 H]NMS) to clarify prerequisites for the analysis of probe signalling. Dualsteric ligands may principally bind in two orientations, the dualsteric mode (pose 1 in Fig. 1c ) and the purely allosteric mode (pose 2 in Fig. 1c ). As receptor activation is encoded by their orthosteric agonist building block, the probes of this study will be agonistic only in the dualsteric posture. Iper-6-naph was chosen for validation of dualsteric binding, because, first, the naphthalimide residue has a higher allosteric M 2 receptor-binding affinity than phthalimide, and, second, the six-membered linker is less suited for an unconstrained dualsteric receptor interaction than the eight-membered linker (see below). Equilibrium and dissociation binding experiments revealed a pronounced preference of iper-6-naph for the dualsteric pose relative to the allosteric pose ( Fig. 2 ). 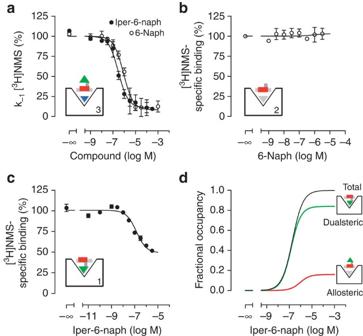Figure 2: Verification of dualsteric probe binding in live CHO-hM2cells. Iper-6-naph is chosen for verification of dualsteric binding in whole cells, because, first, the naph-building block has a higher binding affinity to the allosteric binding area than the phth-binding block and, second, signalling of iper-6-naph is most compromised among all probes, which could theoretically be due to a low probability of dualsteric binding (pose 1). '6-naph' (equivalent to compound 'A2' in ref.24and re-synthesized precisely as described therein) serves as a surrogate for the allosteric building block of iper-6-naph. (a) After having determined radioligand ([3H]NMS)-binding characteristics (pose 4), the affinity of iper-6-naph for the radioligand-bound receptor (pose 3) is derived from probe-induced inhibition of radioligand-dissociation (EC50, diss=α×KB, allo). As to be expected iper-6-naph and 6-naph have almost the same affinity to the [3H]NMS-bound receptor. (b) Interaction of 6-naph with the radioligand under equilibrium binding conditions and analysis based on the ternary complex model is taken to represent the affinity of iper-6-naph for the purely allosteric binding pose 2. (c) Interaction of iper-6-naph with the radioligand under equilibrium conditions and data analysis including binding constants for poses 2 and 3 (modified after55) yields the binding constant for the dualsteric mode (pose 1). (d) The ratio of binding constants for poses 1 and 2 displays the concentration-dependent fractional receptor occupancy of iper-6-naph (black curve) in the dualsteric (green curve, 84%) and allosteric (red curve, 16%) binding mode. Error bars indicate s.e.m. of 6–12 replicates from 2–4 independent experiments. Figure 2: Verification of dualsteric probe binding in live CHO-hM 2 cells. Iper-6-naph is chosen for verification of dualsteric binding in whole cells, because, first, the naph-building block has a higher binding affinity to the allosteric binding area than the phth-binding block and, second, signalling of iper-6-naph is most compromised among all probes, which could theoretically be due to a low probability of dualsteric binding (pose 1). '6-naph' (equivalent to compound 'A2' in ref. 24 and re-synthesized precisely as described therein) serves as a surrogate for the allosteric building block of iper-6-naph. ( a ) After having determined radioligand ([ 3 H]NMS)-binding characteristics (pose 4), the affinity of iper-6-naph for the radioligand-bound receptor (pose 3) is derived from probe-induced inhibition of radioligand-dissociation (EC 50, diss = α × K B, allo ). As to be expected iper-6-naph and 6-naph have almost the same affinity to the [ 3 H]NMS-bound receptor. ( b ) Interaction of 6-naph with the radioligand under equilibrium binding conditions and analysis based on the ternary complex model is taken to represent the affinity of iper-6-naph for the purely allosteric binding pose 2. ( c ) Interaction of iper-6-naph with the radioligand under equilibrium conditions and data analysis including binding constants for poses 2 and 3 (modified after [55] ) yields the binding constant for the dualsteric mode (pose 1). ( d ) The ratio of binding constants for poses 1 and 2 displays the concentration-dependent fractional receptor occupancy of iper-6-naph (black curve) in the dualsteric (green curve, 84%) and allosteric (red curve, 16%) binding mode. Error bars indicate s.e.m. of 6–12 replicates from 2–4 independent experiments. Full size image M 2 receptors prefer coupling to G i over G s proteins [30] , [31] ( Fig. 1c ). Pretreatment of CHO-hM 2 cells with pertussis toxin (PTX) to silence G i - and disclose G s coupling does not affect binding of iper-6-naph and other probes. Binding data are compiled in Supplementary Fig. S1 and Supplementary Table S1 . Dualsteric probes induce structure-dependent G i bias 7TMR proteins can be considered as dynamically fluctuating macromolecules that adopt ensembles of tertiary conformations [5] . Label-free techniques use native receptor proteins thus ensuring natural conformational flexibility and sensitivity to probe actions. Recently, we established dynamic mass redistribution (DMR) as a novel and powerful label-free technology to identify G-protein-dependent signalling in live cells [32] , [33] . Of note, 7TMR signalling along a given pathway may yield cell type-dependent DMR responses [33] . Here, we applied CHO-hM 2 cells. As CHO cells do not generate ACh esterase [34] , they are well suited to quantify DMR responses to the endogenous transmitter ACh ( Fig. 3a–d ). ACh is known to activate G i and G s signalling of M 2 receptors [30] , [31] . Native CHO-hM 2 cells respond to ACh in a concentration-dependent manner with brisk positive DMR ( Fig. 3a ), which suggests G i pathway activation [32] , [33] . Cells pretreated with PTX to chemically knockout G i proteins respond to ACh with negative DMR ( Fig. 3b ). As this signal is completely sensitive to cholera toxin (CTX), which is known to mask G s -mediated signalling [32] , [33] , the negative DMR reflects G s pathway activation ( Supplementary Fig. S2 ). Therefore, positive DMR observed in unpretreated cells includes G i - and G s -mediated signalling events. However, the brisk peak DMR seen in unpretreated cells represents G i activation as, first, this peak is still present in CTX-pretreated cells ( Fig. 3c ) and, second, potencies of ACh for inducing positive peak DMR in the absence and presence of CTX are in the same range ( Fig. 3d , control: pEC 50 =8.09±0.13; CTX: pEC 50 =7.49±0.16; P =0.02, unpaired t -test). The small, albeit significant, difference in potencies is likely to be caused by cellular adaptation to the CTX-induced rise of intracellular cyclic AMP (cAMP). In contrast, the potency of ACh for G s activation (pEC 50 =6.01±0.19) is 100-fold lower compared with positive peak DMR and 30-fold lower relative to positive peak DMR in CTX-pretreated cells ( P <0.001, one-way analysis of variance (ANOVA) with Dunnett's post test). Taken together, peak DMR in unpretreated cells represents G i activation. 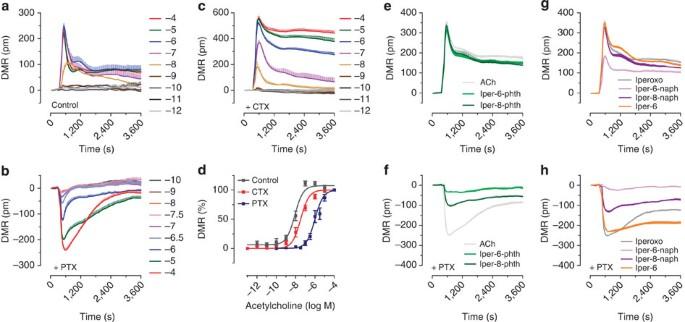Figure 3: Cellular DMR reveals structure-dependent Gibias of dualsteric probes. (a–c) Shown are baseline-corrected DMR responses measured as wavelength shifts (pm) and recorded over time after addition of indicated concentrations of ACh in non-pretreated CHO-hM2cells (control,a) and either PTX (b)- or CTX (c)-pretreated CHO-hM2cells (means and s.e.m.) from one representative out of at least four independent experiments conducted in quadruplicates. (a) ACh exposure of control cells induces concentration-dependent positive DMR with peaks reflecting Gisignalling. (b) Pretreatment with the Giinhibitor PTX (100 ng ml−1, 16–24 h) reveals negative DMR reflecting Gssignalling. (c) Masking Gs-dependent signalling by CTX pretreatment (100 ng ml−1, 8 h) induces positive DMR followed by sustained plateaus at higher concentrations. (d) Concentration-effect curves of ACh-induced peak DMR; data (means±s.e.m. from at least four experiments) are normalized to the response obtained with 100 μM ACh. The pronounced sensitivity of ACh's potency to PTX indicates Gidominance in the control DMR peaks. (e–h) DMR recordings of indicated compounds in either control cells (e,g) or PTX-pretreated cells (f,h). Applied were maximally effective concentrations: ACh 100 μM, iper-6-phth 100 μM, iper-8-phth 10 μM, iperoxo 1 μM, iper-6-naph 100 μM, iper-8-naph 10 μM and iper-6 100 μM. Representative data (means and s.e.m.) of at least three independent experiments conducted in quadruplicates. Figure 3: Cellular DMR reveals structure-dependent G i bias of dualsteric probes. ( a – c ) Shown are baseline-corrected DMR responses measured as wavelength shifts (pm) and recorded over time after addition of indicated concentrations of ACh in non-pretreated CHO-hM 2 cells (control, a ) and either PTX ( b )- or CTX ( c )-pretreated CHO-hM 2 cells (means and s.e.m.) from one representative out of at least four independent experiments conducted in quadruplicates. ( a ) ACh exposure of control cells induces concentration-dependent positive DMR with peaks reflecting G i signalling. ( b ) Pretreatment with the G i inhibitor PTX (100 ng ml −1 , 16–24 h) reveals negative DMR reflecting G s signalling. ( c ) Masking G s -dependent signalling by CTX pretreatment (100 ng ml −1 , 8 h) induces positive DMR followed by sustained plateaus at higher concentrations. ( d ) Concentration-effect curves of ACh-induced peak DMR; data (means±s.e.m. from at least four experiments) are normalized to the response obtained with 100 μM ACh. The pronounced sensitivity of ACh's potency to PTX indicates G i dominance in the control DMR peaks. ( e – h ) DMR recordings of indicated compounds in either control cells ( e , g ) or PTX-pretreated cells ( f , h ). Applied were maximally effective concentrations: ACh 100 μM, iper-6-phth 100 μM, iper-8-phth 10 μM, iperoxo 1 μM, iper-6-naph 100 μM, iper-8-naph 10 μM and iper-6 100 μM. Representative data (means and s.e.m.) of at least three independent experiments conducted in quadruplicates. Full size image Dualsteric probes exhibit a G i over G s signalling bias compared with ACh and iperoxo ( Fig. 3e–h ), which induce equieffective promiscous G i and G s signalling (compare DMR peaks in Fig. 3 , panels e with g and f with h, respectively). Noteworthy, pretreatment with PTX did not affect receptor density ( B max -PTX=89% of B max -control, P =0.75, unpaired t -test). Relative to these agonists, iper-6 has comparable maximum effects ( Fig. 3g,h ). In contrast, iper-6-phth and iper-8-phth, although being almost equieffective to orthosteric agonists with respect to G i -DMR ( Fig. 3e ), hardly induce G s -DMR ( Fig. 3f ). Of note, the middle chain-elongated iper-8-phth is more competent for G s -DMR than iper-6-phth ( Fig. 3f ). In case of the spacious iper-x-naph analogues, even G i -DMR is compromised with iper-6-naph ( Fig. 3g ), whereas the middle chain-elongated iper-8-naph clearly achieves maximum G i -DMR ( Fig. 3g ). As found with iper-x-phth analogues, G s -DMR is more compromised than G i -DMR, especially in case of iper-6-naph ( Fig. 3h ) where G s signalling is virtually silenced. Iper-8-naph only partially activates the Gs pathway ( Fig. 3h ), comparable to iper-8-phth ( Fig. 3f ). Peak DMR-values are enumerated in Supplementary Table S2 . Taken together, the DMR findings reveal that G s pathway activation by the hM 2 receptor is far more sensitive to spacious allosteric substituents than G i activation. In addition, probes indicate that the position of the spacious allosteric substituent within the extracellular binding cleft of the receptor protein is crucial for signalling. Quantification of the probes' G i bias DMR measurements point to a structure-dependent signalling bias. We used standard G i and G s signalling readouts that are close downstream to receptor activation for quantifying the probes' signalling bias. [ 35 S]GTPγS binding in membrane suspensions of CHO-hM 2 cells reflects replacement of GDP by GTP at G protein α subunits as a consequence of receptor activation ( Fig. 4a ). This assay almost exclusively captures G i activation [35] . Intracellular cAMP formation in probe-activated CHO-hM 2 cells pretreated with PTX displays activation of the G s pathway ( Fig. 4b ). 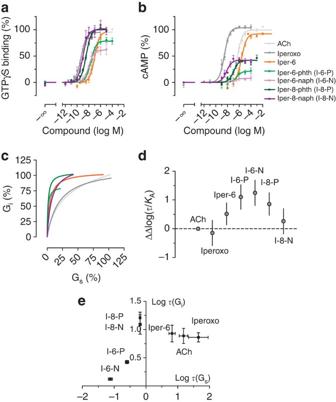Figure 4: Quantifying the Gibias of dualsteric probes. (a) M2receptor-mediated Giprotein activation is reflected by [35S]GTPγS binding to membranes of CHO-hM2cells. Maximum G-protein activation induced by ACh was set 100%. Data are means±s.e.m. from at least four independent experiments conducted in quadruplicates. (b) M2receptor-mediated Gsactivation is reflected by an increase of intracellular cAMP in CHO-hM2cells pretreated with PTX (50 ng ml−1, 16–24 h). Maximum cAMP formation induced by ACh was set 100%. Data are means±s.e.m. from at least three independent experiments conducted in quadruplicates. Concentration-effect curves were obtained by global fits applying the operational model of agonism37to the data points inaandb. (c) Visualization of ligand bias: fractional [35S]GTPγS binding and cAMP accumulation (a,b) are plotted for equal concentrations of the respective agonists on the ordinate and abcissa, respectively. The hyperbolic shape of the ACh graph indicates system bias. The Giprotein is preferred by the M2receptor. Ligands whose bias exceeds system bias display graphs that differ substantially in their curvature radii and the height of their plateaus. (d) Quantification of ligand bias: ΔΔlog(τ/KA) values compensate for system bias and display true ligand bias relative to Ach, which is taken as balanced agonist. Ligands with positive values are Gibiased when the limits of their 95% confidence intervals (CIs) do not contain zero. Data are means with 95% CIs. (e) Efficacies of the agonist-occupied receptor to activate the Gipathway (logτ(Gi)) and the Gspathway (logτ(Gs)) are plotted on the ordinate and abcissa, respectively. Logτvalues are derived from global fits applying the operational model to the data points inaandb. Data are means±s.e.m. Figure 4: Quantifying the G i bias of dualsteric probes. ( a ) M 2 receptor-mediated G i protein activation is reflected by [ 35 S]GTPγS binding to membranes of CHO-hM 2 cells. Maximum G-protein activation induced by ACh was set 100%. Data are means±s.e.m. from at least four independent experiments conducted in quadruplicates. ( b ) M 2 receptor-mediated G s activation is reflected by an increase of intracellular cAMP in CHO-hM 2 cells pretreated with PTX (50 ng ml −1 , 16–24 h). Maximum cAMP formation induced by ACh was set 100%. Data are means±s.e.m. from at least three independent experiments conducted in quadruplicates. Concentration-effect curves were obtained by global fits applying the operational model of agonism [37] to the data points in a and b . ( c ) Visualization of ligand bias: fractional [ 35 S]GTPγS binding and cAMP accumulation ( a , b ) are plotted for equal concentrations of the respective agonists on the ordinate and abcissa, respectively. The hyperbolic shape of the ACh graph indicates system bias. The G i protein is preferred by the M 2 receptor. Ligands whose bias exceeds system bias display graphs that differ substantially in their curvature radii and the height of their plateaus. ( d ) Quantification of ligand bias: ΔΔlog( τ / K A ) values compensate for system bias and display true ligand bias relative to Ach, which is taken as balanced agonist. Ligands with positive values are G i biased when the limits of their 95% confidence intervals (CIs) do not contain zero. Data are means with 95% CIs. ( e ) Efficacies of the agonist-occupied receptor to activate the G i pathway (log τ (G i )) and the G s pathway (log τ (G s )) are plotted on the ordinate and abcissa, respectively. Log τ values are derived from global fits applying the operational model to the data points in a and b . Data are means±s.e.m. Full size image Regarding maximum effects, Fig. 4a,b shows—as observed in the DMR measurements—that iper-6-phth and even more so iper-6-naph are compromised with respect to the G s assay relative to the G i assay. Again, the middle chain-elongated derivatives show increased efficacy for G s signalling ( Fig. 4a,b and Supplementary Table S3 ). The bias plot [36] ( Fig. 4c ) compares signalling via the G i and G s route at equal concentrations of test compound over the range of applied concentrations. The respective maximum effects of ACh define 100%. The hyperbolic curve of ACh reflects its preference for G i activation, which is designated as system bias. Relative to this system bias, all test compounds, except iperoxo, reveal a stronger G i bias. On the receptor level, this may result from a higher affinity ratio of binding to G i - versus G s -coupled receptors. In addition or alternatively, the efficacy τ of an agonist-bound receptor may be higher for signalling via the G i instead of the G s pathway. Global fitting of the functional data ( Fig. 4a,b ) with the operational model of agonism [37] provides measures for both the binding constant ( K A ) and the efficacy ( τ ) of the respective agonists. The τ / K A -ratio [38] (transduction coefficient) encompasses both potential mechanisms of bias (for τ / K A -ratios for both pathways normalized on ACh (Δlog( τ / K A )) see Table 1 ). ΔΔlog(τ/ K A )-values [38] ( Fig. 4d , Table 1 ) eliminate system bias and indicate true test compound bias relative to ACh. In general, dualsteric agonists are significantly G i biased ( Fig. 4d ). Iper-8-naph is an exception; this compound has clearly lower efficacy on the G s pathway ( Fig. 4b ) than ACh, which, however, is compensated by a higher binding affinity (low K A -value; Supplementary Table S4 ). Figure 4e focusses on the efficacy component of ligand bias. Plotted is the efficacy log τ of agonist-bound receptors for activating G i and G s signalling. The iper-6-naph-bound receptor has lowest signalling efficacy. The latter is restored by replacement of the naph-residue by the less voluminous phth-residue and even more by linker elongation from C6 to C8. Iper-8-naph and iper-8-phth attain an upper level of G i activation, which is not surpassed by ACh and iperoxo, but are still clearly inferior with respect to G s activation. Shortening of the dualsteric agonists to iper-6 and further to iperoxo then stepwise restores G s signalling efficacy. These findings corroborate the notion that G s signalling efficacy of the agonist-bound M 2 receptor is more sensitive to the allosteric residues of dualsteric probes than G i signalling efficacy ( Supplementary Table S4 ). Table 1 Parameters characterizing ligand bias of muscarinic agonists. Full size table Middle chain elongation restores signalling at different levels As 7TMR ligands may have widely differing signalling competence depending on pathways (for review see refs 39 , 40 ), we investigated the probes' signalling pattern in a set of additional readouts. First, we focused on the receptor's intracellular loops, as these mediate receptor contact with adaptor proteins. We used a FRET-sensor-hM 2 -receptor, stably expressed in HEK293 cells, that has an enhanced cyan fluorescent protein (eCFP) fused to its C-terminus and a FlAsH-binding domain introduced within the third intracellular loop beneath transmembrane domain TM5, respectively [41] , [42] , [43] , [44] ( Supplementary Methods ). Agonist-induced conformational transitions of the inner loop region were diminished in the case of iper-6 and not significantly different from baseline in the case of iper-6-phth and iper-6-naph ( Fig. 5a ). Intracellular loop movements reappeared with the iper-8-X compounds. Thus, the allosteric substituents introduced into the orthosteric iperoxo and pointing to the extracellular surface of the receptor protein severely restrict inner loop region dynamics. Noteworthy, shifting the spacious residues further outward in the allosteric region by middle chain elongation unleashes orthosteric agonist-like intracellular loop rearrangement. 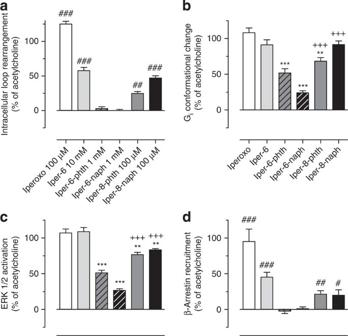Figure 5: M2receptor inner loop and adaptor protein rearrangement and downstream signalling. (a) Intracellular loop rearrangement on receptor activation was determined as a change in FRET in HEK293 cells transfected to stably express a N-FLAG-tagged hM2FlAsH–eCFP fusion protein. Maximum FRET induced by 100 μM ACh was set 100%. Data are means and s.e.m. from 12–15 cells of at least three independent experiments. (b) M2receptor-mediated conformational change of the Gαi-subunit relative to the βγ-subunit was measured as an indicator of G-protein activation in COS-7 cells transfected to transiently coexpress the hM2receptor, Gαi1-91Rluc and GFP10-Gγ2along with the complementary subunit Gβ1. Maximum BRET on ACh exposure (100 μM) was set 100%. Data are means and s.e.m. from at least four independent experiments. (c) M2receptor-mediated ERK1/2 activation was assessed in live CHO-hM2cells using a htrf-based sandwich immunoassay. Maximum FRET induced by 100 μM ACh was set 100%. Data are means and s.e.m. from four independent experiments. (d) β-Arrestin recruitment on M2receptor activation was captured in a BRET-based proximity assay using a stable HEK-293-GFP2-β-arr2 cell line transfected to transiently coexpress the hM2receptor–Rluc fusion protein and GRK2. Ligand-promoted BRET was normalized to 100 μM ACh. Data are means and s.e.m. from at least three independent experiments. Applied ligand concentrations—unless indicated otherwise—were 100 μM except for iperoxo 1 μM, iper-8-phth 10 μM and iper-8-naph 10 μM., (***P<0.001,**P<0.01) significantly different from ACh 100 μM, (+++P<0.001) significantly different from iper-6-phth and iper-6-naph, respectively, (###P<0.001,##P<0.01,#P<0.05) significantly different from vehicle according to one-way ANOVA and Bonferroni's multiple comparison test. Figure 5: M 2 receptor inner loop and adaptor protein rearrangement and downstream signalling. ( a ) Intracellular loop rearrangement on receptor activation was determined as a change in FRET in HEK293 cells transfected to stably express a N-FLAG-tagged hM 2 FlAsH–eCFP fusion protein. Maximum FRET induced by 100 μM ACh was set 100%. Data are means and s.e.m. from 12–15 cells of at least three independent experiments. ( b ) M 2 receptor-mediated conformational change of the Gα i -subunit relative to the βγ-subunit was measured as an indicator of G-protein activation in COS-7 cells transfected to transiently coexpress the hM 2 receptor, Gα i1 -91Rluc and GFP10-Gγ 2 along with the complementary subunit Gβ 1 . Maximum BRET on ACh exposure (100 μM) was set 100%. Data are means and s.e.m. from at least four independent experiments. ( c ) M 2 receptor-mediated ERK1/2 activation was assessed in live CHO-hM 2 cells using a htrf-based sandwich immunoassay. Maximum FRET induced by 100 μM ACh was set 100%. Data are means and s.e.m. from four independent experiments. ( d ) β-Arrestin recruitment on M 2 receptor activation was captured in a BRET-based proximity assay using a stable HEK-293-GFP 2 -β-arr2 cell line transfected to transiently coexpress the hM 2 receptor–Rluc fusion protein and GRK2. Ligand-promoted BRET was normalized to 100 μM ACh. Data are means and s.e.m. from at least three independent experiments. Applied ligand concentrations—unless indicated otherwise—were 100 μM except for iperoxo 1 μM, iper-8-phth 10 μM and iper-8-naph 10 μM., ( *** P <0.001, ** P <0.01) significantly different from ACh 100 μM, ( +++ P <0.001) significantly different from iper-6-phth and iper-6-naph, respectively, ( ### P <0.001, ## P <0.01, # P <0.05) significantly different from vehicle according to one-way ANOVA and Bonferroni's multiple comparison test. Full size image Next, we examined conformational transitions of the G i protein ( Fig. 5b and Supplementary Methods ). Therefore, the activation-promoted rearrangement of the α-subunit relative to the βγ-subunit was analysed using a protein–protein-interaction-based bioluminescence resonance energy transfer (BRET) assay [45] in COS7-cells. These were transiently co-transfected with the hM 2 receptor and the Renilla luciferase-tagged Gα i 1-subunit along with Gβ and a GFP-tagged γ-subunit. All probes induce a conformational rearrangement of the G i protein with the iper-8-X compounds displaying a higher efficacy than the respective iper-6-X probes. Compared with the inner loop-assay ( Fig. 5a ), efficacies are generally higher, which is likely due to a receptor reserve in the latter assay. Taken together, restricted capacity of the dualsteric probes for inducing inner loop rearrangement translates into diminished G-protein activation. ERK1/2 phosphorylation is triggered by the βγ-subunit of active G i proteins [46] . The active βγ-subunit directly interacts with phosphoinositide 3-kinase γ inducing a series of downstream events resulting in increased ERK1/2-phosphorylation and eventually in modified gene expression [47] . M 2 receptor-mediated ERK1/2-phosphorylation in CHO cells is exclusively G i -dependent, as it is completely abolished after PTX pretreatment ( Supplementary Fig. S3 ). As iper-6-X compounds are less efficacious than their middle chain-elongated iper-8-X fellows ( Fig. 5c ), the structure-dependent efficacy pattern is similar to that encountered in G i readouts ( Figs 3e,g and 4a ). β-Arrestin recruitment was studied in HEK293 cells stably expressing GFP-β-arrestin2 and transiently coexpressing the hM 2 –Rluc fusion protein and GRK2 ( Supplementary Methods ). The construct has full signalling competence with respect to G i and G s signalling ( Supplementary Fig. S4 ). β-Arrestin recruitment is partially restored in the middle chain-elongated derivatives iper-8-X relative to the hexamethylene compounds iper-6-X ( Fig. 5d ). Taken together, dualsteric probe-induced reduction of the receptor's allosteric domain flexibility translates into restricted intracellular loop rearrangement and, subsequently, to impaired downstream signalling events. An allosteric space 'rescue mutation' boosts signalling In order to further test the hypothesis that M 2 receptor signalling critically depends on a conformational narrowing in the core region of the receptor's allosteric vestibule near M 2 -W422 7.35 , we replaced the spacious tryptophan by the small alanine. This should unleash signalling of the dualsteric agonists. We focused on iper-6-phth and iper-6-naph, as these probes displayed the weakest signalling efficacy in the preceding experiments. M 2 -W422 7.35 A reduces binding affinities of ACh ( Fig. 6a ) and iperoxo ( Fig. 6b ). The respective potencies for G-protein activation are diminished to the same extent ( Fig. 6c,d ). Both, iper-6-phth and iper-6-naph lose binding affinity and, to a lesser extent, potency at mutant receptors ( Fig. 6a–d and Supplementary Table S5 ). Most importantly, the allosteric mutation leads to a gain in dualsteric probes' efficacy ( Fig. 6c,d ). As the surface expression of mutant receptors was about one-third lower compared with wild type ( Supplementary Fig. S5 ), evaluation based on maximum effects would even underestimate the ligand's true capacity for receptor activation. Comparison of log τ -values reveals that efficacy for G i activation of iper-6-phth and iper-6-naph in the mutant are indistinguishable from that of iperoxo ( Fig. 6e ). 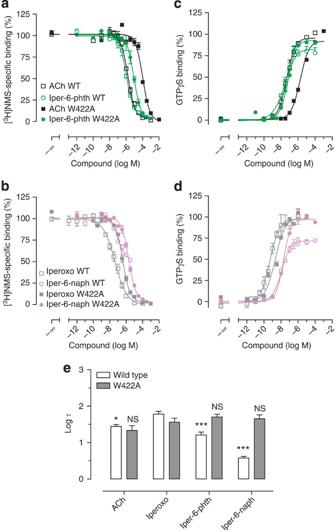Figure 6: Recovery of Gisignalling of dualsteric probes in the allosteric M2W4227.35A receptor mutant. (a,b) Equilibrium cell surface receptor binding of ACh, iperoxo, iper-6-phth and iper-6-naph competing against [3H]NMS in live CHO-hM2cells (open symbols) and CHO-hM2W4227.35A cells (filled symbols). Data are means±s.e.m. from at least three independent experiments conducted in triplicates. Binding curve fitting was based either on the four-parameter logistic function or on the allosteric ternary complex model in case of iper-6-phth wild type (WT) and iper-6-naph WT. Binding constants for the M2WT receptor and M2W422A mutant receptor were 5.86±0.04 and 4.36±0.02 for ACh, 7.49±0.16 and 6.81±0.01 for iperoxo, 6.11±0.06 and 5.45±0.09 for iper-6-phth and 7.07±0.08 and 6.05±0.04 for iper-6-naph, respectively. (c,d) M2receptor-mediated Giprotein activation was measured as reflected by [35S]GTPγS binding to membranes of CHO-hM2cells (open symbols) and CHO-hM2W4227.35A cells (filled symbols). Maximum G-protein activation induced by ACh was set 100%. Data are means±s.e.m. from at least three independent experiments conducted in quadruplicates. Curve fitting incanddwas based on the operational model of agonism using the ligand-binding affinities derived fromaandb. (e) Coupling efficiencies of indicated ligands at the M2WT receptor and the M2W4227.35A receptor mutant. (***P<0.001,*P<0.05), significantly different from iperoxo at the M2WT receptor according to two-way ANOVA with Bonferroni's multiple comparison test, NS, not significantly different from iperoxo at the mutant receptors. Figure 6: Recovery of G i signalling of dualsteric probes in the allosteric M 2 W422 7.35 A receptor mutant. ( a , b ) Equilibrium cell surface receptor binding of ACh, iperoxo, iper-6-phth and iper-6-naph competing against [ 3 H]NMS in live CHO-hM 2 cells (open symbols) and CHO-hM 2 W422 7.35 A cells (filled symbols). Data are means±s.e.m. from at least three independent experiments conducted in triplicates. Binding curve fitting was based either on the four-parameter logistic function or on the allosteric ternary complex model in case of iper-6-phth wild type (WT) and iper-6-naph WT. Binding constants for the M 2 WT receptor and M 2 W422A mutant receptor were 5.86±0.04 and 4.36±0.02 for ACh, 7.49±0.16 and 6.81±0.01 for iperoxo, 6.11±0.06 and 5.45±0.09 for iper-6-phth and 7.07±0.08 and 6.05±0.04 for iper-6-naph, respectively. ( c , d ) M 2 receptor-mediated G i protein activation was measured as reflected by [ 35 S]GTPγS binding to membranes of CHO-hM 2 cells (open symbols) and CHO-hM 2 W422 7.35 A cells (filled symbols). Maximum G-protein activation induced by ACh was set 100%. Data are means±s.e.m. from at least three independent experiments conducted in quadruplicates. Curve fitting in c and d was based on the operational model of agonism using the ligand-binding affinities derived from a and b . ( e ) Coupling efficiencies of indicated ligands at the M 2 WT receptor and the M 2 W422 7.35 A receptor mutant. ( *** P <0.001, * P <0.05), significantly different from iperoxo at the M 2 WT receptor according to two-way ANOVA with Bonferroni's multiple comparison test, NS, not significantly different from iperoxo at the mutant receptors. Full size image Probe-induced maximum DMR was compared between CHO-hM 2 cells ( Fig. 7a,b ) and CHO-hM 2 -W422 7.35 A cells ( Fig. 7b,c ). Both, PTX pretreatment and the allosteric mutation lead to a pronounced loss of orthosteric agonist potency ( Figs 3d and 6c,d ). Under these conditions, iperoxo—due to its high potency—still achieves a clear maximum effect on the G s pathway at the mutant receptor and was therefore used instead of ACh to define full efficacy and balanced agonism (for original DMR traces see Supplementary Fig. S6 ). As reported above ( Fig. 6 and Supplementary Table S5 ), dualsteric probe potency is little affected by the mutation. Probes were applied at maximally effective concentrations with respect to both, G s and G i pathway activation. Under these conditions, maximum effects can be taken to reflect coupling efficacy τ . In the mutant receptor, maximum G s -DMR induced by the probes is increased in case of the iper-6-X compounds and iper-8-phth ( Fig. 7b ). Only in the case of iper-8-naph, which has the highest G s -DMR among the dualsteric probes at wild-type hM 2 receptor, a further increase in maximum G s -DMR was not observed. The most impressive gain in G s pathway activation is found with iper-8-phth, yet full G s signalling is not achieved in the mutant ( Fig. 7b,c ). As mentioned previously ( Fig. 6 ), the mutant receptor also allows for a gain in efficacy for G i signalling, which is most pronounced for iper-6-naph (see ordinates in Fig. 7a,c ). 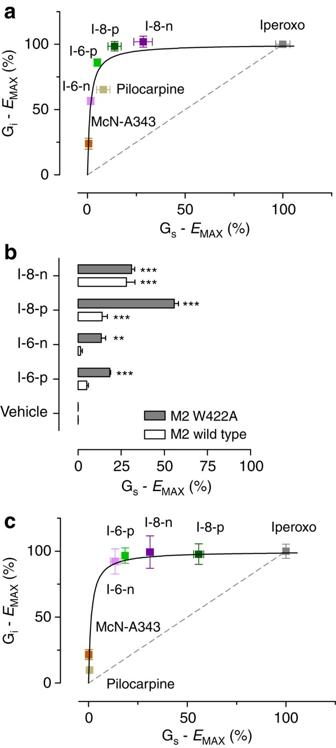Figure 7: Gssignalling of dualsteric probes is augmented in the W4227.35A mutant. (a,c) Maximum Gi- and Gs-DMR effects of the indicated compounds in wild-type CHO-hM2cells (a) or CHO-hM2W4227.35A cells (c). Data represent means±s.e.m. from three independent experiments inaandc. Cells were pretreated with PTX 100 ng ml−1for 16–24 h to disclose Gssignalling. All concentrations used provide maximum effects for both the Giand the Gspathway according to GTPγS binding and cAMP accumulation assays, respectively. Data were normalized on the respective effect of iperoxo 10 μM, which was set 100% for each condition. Dashed lines represent balanced agonism. Continuous lines define a binodal curve resulting from a best fit to the indicated data points ina. Concentrations of ligands: iperoxo 10 μM, iper-6-phth (i-6-p) 100 μM, iper-8-phth (i-8-p) 10 μM, iper-6-naph (i-6-n) 100 μM, iper-8-naph (i-8-n) 10 μM, pilocarpine 100 μM and McN-A-343 100 μM. (b) Iper-6-phth and iper-6-naph induce significant Gssignalling at the hM2W4227.35A mutant in contrast to wild-type receptors. Shown are maximal DMR responses normalized to the DMR of iperoxo 10 μM (set 100%) in CHO-hM2cells (wild type, open bars) and CHO-hM2W4227.35A cells (filled bars). Data are means±s.e.m of at least three independent experiments. *P<0.05,**P<0.01, ***P<0.001, significant to vehicle according to a two-way ANOVA with Bonferroni's multiple comparison test. Figure 7: G s signalling of dualsteric probes is augmented in the W422 7.35 A mutant. ( a , c ) Maximum G i - and G s -DMR effects of the indicated compounds in wild-type CHO-hM 2 cells ( a ) or CHO-hM 2 W422 7.35 A cells ( c ). Data represent means±s.e.m. from three independent experiments in a and c . Cells were pretreated with PTX 100 ng ml −1 for 16–24 h to disclose G s signalling. All concentrations used provide maximum effects for both the G i and the G s pathway according to GTPγS binding and cAMP accumulation assays, respectively. Data were normalized on the respective effect of iperoxo 10 μM, which was set 100% for each condition. Dashed lines represent balanced agonism. Continuous lines define a binodal curve resulting from a best fit to the indicated data points in a . Concentrations of ligands: iperoxo 10 μM, iper-6-phth (i-6-p) 100 μM, iper-8-phth (i-8-p) 10 μM, iper-6-naph (i-6-n) 100 μM, iper-8-naph (i-8-n) 10 μM, pilocarpine 100 μM and McN-A-343 100 μM. ( b ) Iper-6-phth and iper-6-naph induce significant G s signalling at the hM 2 W422 7.35 A mutant in contrast to wild-type receptors. Shown are maximal DMR responses normalized to the DMR of iperoxo 10 μM (set 100%) in CHO-hM 2 cells (wild type, open bars) and CHO-hM 2 W422 7.35 A cells (filled bars). Data are means±s.e.m of at least three independent experiments. * P <0.05,** P <0.01, *** P <0.001, significant to vehicle according to a two-way ANOVA with Bonferroni's multiple comparison test. Full size image The partial agonists pilocarpine and McN-A-343 are included in Fig. 7 for comparison. Pilocarpine has an orthosteric binding topography [29] , McN-A-343 is a bitopic allosteric/orthosteric partial agonist at hM 2 receptors [48] . Pilocarpine and McN-A-343 respond differently to the mutation compared with the dualsteric probes ( Fig. 7a,c ), as the efficacy of pilocarpine is almost completely lost, whereas the efficacy of McN-A-343 does not differ from hM 2 wild type (all E max values are enumerated in Supplementary Table S6 ). These findings underpin that the dualsteric probes exhibit a unique molecular mechanism of receptor interaction. Importantly, the increase in G i /G s signalling of the dualsteric compounds in CHO-hM 2 -W422 7.35 A cells ( Fig. 7c ) strictly follows the hyperbolic relationship defined for CHO-hM 2 cells ( Fig. 7a ). Obviously, nearly full efficacy for G i signalling is required before additional G s signalling can emerge. We conclude that the receptor conformation mediating G s signalling is reached via an intermediate conformation, the signalling efficacy of which is confined to G i activation. In recent years, accumulating evidence suggests that signalling promiscuity is a general principle of 7TMR biology. For many 7TMRs, ligands are available that selectively activate a subset of signalling pathways [3] , [40] . The mechanisms underlying multiple signalling pathway activation and functional selectivity are far from being understood [12] . Applying a new methodological approach, this study provides hitherto unprecedented insights into the role of the allosteric vestibule for the discrimination between signalling pathways of a 7TMR. In order to allow for the subtle conformational transitions that underlie signalling promiscuity and selectivity [8] , we laid emphasis on the study of a native, unlabelled receptor protein. To probe the role of the receptor's extracellular domain for discriminating signalling pathway activation, we applied small molecules designed to interfere in a graded manner with activation-related extracellular domain rearrangements. Our study shows that this strategy allows capturing conformational dynamics underlying differential signalling pathway activation. Several studies show that extracellular loops, especially the second extracellular loop, take part in the binding and activation of rhodopsin-like class A 7TMRs [49] . Until now, however, the molecular events have not been elucidated by which the extracellular region is functionally linked with the intracellular control of adaptor protein recruitment and the consecutive differential activation of signalling pathways. Here we show for the first time that relay of signalling triggered by orthosteric agonist binding critically depends on spatial freedom for concurrent extracellular conformational transitions. Allosteric substituents—attached to the orthosteric agonist iperoxo—that protrude into the free volume of the extracellular loop region severely hamper signalling of the M 2 receptor. Structure–activity relationships of dualsteric probes and employment of the hM 2 -W422 7.35 A mutant receptor allowed to narrow down a critical region of the M 2 receptor in the vicinity of W422 7.35 , which is located above the orthosteric-binding pocket at the contact between the third extracellular loop and the beginning of TM7 (ref. 25 ). This epitope is conserved among the five subtypes of the muscarinic receptor. M 2 -W422 7.35 has been suggested to form a link with M 2 -Y177 5.32 of the second extracellular loop and to undergo a conformational rearrangement on receptor activation [29] . Interestingly, comparison of the crystal structures of the inactive and the active β 2 receptor revealed that receptor activation involves a movement of the corresponding β 2 -Y308 7.35 towards β 2 -F193 5.32 of the second extracellular loop, thereby narrowing the free volume above the orthosteric site [10] . Our strategy of probing conformational freedom including the 'rescue mutant' M 2 W422 7.35 A demonstrates that the corresponding region of the M 2 receptor is critical for G-protein coupling. The physiological function of allosteric binding areas of class A 7TMR is only beginning to be understood. Evidence for a mechanism of general importance has recently been provided for β 1 and β 2 adrenergic receptors. Molecular dynamics simulations imply that ligand entry into and exit from the orthosteric site is a two-step event that includes intermediate ligand binding to a vestibule formed in the receptor's extracellular domains [50] , [51] . The first step, entry into the vestibule, appears to be important for the removal of water molecules from the ligand [50] . The subsequent passage leading from the allosteric vestibule into the orthosteric-binding cavity of the β 2 receptor is lined by β 2 -Y308 7.35 and β 2 -F193 5.32 (ref. 50 ). As these epitopes are rearranged in the course of the inactive-to-active receptor transition [10] , it is likely that this rearrangement occurs parallel to or is even caused by the ligand moving along the passage into the orthosteric site. Our findings disclose that spatial rearrangement of this passage in the M 2 receptor is critical for receptor movements required for appropriate unfolding of the intracellular domain region for G-protein coupling. In particular, we show that the allosteric vestibule of the muscarinic M 2 receptor has to provide room for a 'standard' conformational rearrangement allowing G i coupling and an 'extended' movement for G s coupling. Beyond that we show that the G s activation-competent receptor conformation is reached via an intermediate conformation with full efficacy for G i activation. Hence, for the first time we assign a biological role to the allosteric vestibule for controlling G-protein signalling of a 7TMR. Crystal structures of active class A 7TMRs point to a common activation mechanism including cytosolic outwards movement of transmembrane helices and a corresponding inwards movement of extracellular domains [9] , [10] , [11] . In the end, the novel chemical–biological strategy introduced here offers a widely applicable label-free approach for clarifying the dependence of promiscuous signalling pathway activation on extracellular domain rearrangements. This does not only apply to 7TMRs that are already known to bind allosteric or even dualsteric ligands [52] . The new strategy will be of even broader relevance if the extracellular vestibule-mediated ligand-binding process represents a more general mechanism [50] , [51] . With respect to drug discovery, our findings likely disclose a general route for the design of a new type of biased agonist. It is unique as it addresses two distinct receptor sites simultaneously with opposing functional messages, that is activation of the orthosteric receptor region by the agonist moiety and inactivation of an allosteric domain by an antagonist or even inverse agonist moiety [29] , [53] . When applied un-tethered, the components reveal strong negative binding cooperativity as previously shown with orthosteric ACh and allosteric naph- or phth-residues [29] reflecting a severe conformational mismatch. On covalent linkage of these building blocks, dualsteric binding is enforced leading to a receptor conformation, which is unlikely to occur with un-tethered ligands and has specific signalling properties. The choice of building blocks and linker-length allows designing custom-made receptor activators endowed with desired signalling phenotypes. We conclude that the allosteric vestibule serves to fine-tune the nature of signals generated on orthosteric ligand activation of a 7TMR. The activation of differential signalling pathways piloted by extracellular domains is due to sequential conformational states of the receptor protein and eventually results in a hierarchical order of intracellular adaptor protein recruitment. As several family A 7TMRs harbour an allosteric vestibule within their outer domains, the findings also suggest that controlling G-protein coupling is a general biological role of 7TMR allosteric vestibules. Cell culture Flp-In-Chinese hamster ovary cells (Flp-In-CHO) stably expressing the hM 2 receptor (CHO-hM 2 cells) or the hM 2 W422A mutant receptor (CHO-hM 2 W422A cells) and CHO-K1 cells were cultured in Ham's nutrient mixture F-12 supplemented with 10% (v/v) fetal calf serum (FCS), 100 U ml −1 penicillin, 100 μg ml −1 streptomycin and 2 mM L -glutamine. COS-7 cells were grown in DMEM supplemented with 10% (v/v) FCS, 100 U ml −1 penicillin and 100 μg ml −1 streptomycin. HEK293 cell clones stably expressing either GFP2-β-arr2 or the hM 2 receptor FRET-sensor, respectively, were maintained in DMEM supplemented with 10% (v/v) FCS, 100 U ml −1 penicillin, 100 μg ml −1 streptomycin and 200–500 μg ml −1 G418. All cell lines were kept at 37 °C in a humidified 5% CO 2 atmosphere (7% CO 2 for HEK293 cells stably expressing the hM2 FRET-sensor). Radioligand-binding assay CHO-hM 2 and CHO-hM 2 W422A cells were seeded on cell culture dishes and grown for 2 days. For PTX experiments, cells were pretreated with PTX (100 ng ml −1 ) for 16–24 h before the assay. Cells were collected and adjusted to give a final concentration of 750,000 cells per ml in assay buffer (Hank's balanced salt solution (HBSS) supplemented with 20 mM HEPES; pH 7.0). All experiments were carried out with 75,000 cells per well in a 96-well microtiterplate (Abgene, Germany) at 28 °C in a final volume of 500 μl. Experiments were terminated by rapid vacuum filtration and bound radioactivity was determined by solid scintillation counting. For two-point kinetic dissociation experiments, cells were pre-incubated with 2 nM [ 3 H]NMS for 45 min before addition of dualsteric compounds. Reassociation of [ 3 H]NMS was prevented by 10 μM atropine and reactions were terminated after 10 min. For equilibrium binding experiments, cells were incubated for 4 h with 0.2 nM [ 3 H]NMS and agonists at different concentrations to reach equilibrium. To make sure that binding equilibrium was attained in presence of dualsteric compounds, incubation time was calculated as described previously [23] . DMR assay DMR assays were performed on a beta version of the Corning Epic biosensor. A detailed protocol is published elsewhere [33] . Briefly, CHO-hM 2 wild-type, CHO-hM 2 W422A cells and CHO-K1 cells transfected to transiently express the hM 2 wild-type receptor or a FLAG-tagged hM 2 receptor–Rluc fusion protein were grown to confluence for 20–24 h on Epic biosensor 384-well microplates. Cells were washed twice with HBSS containing 20 mM HEPES (pH 7.0) and kept for 2 h in the Epic reader at 28 °C. DMR was monitored before (baseline read) and after the addition of compound solutions for 3,600 s. Pre-incubation time for CTX (100 ng ml −1 ) pretreatment and PTX (100 ng ml −1 ) pretreatment was 8 and 16–24 h, respectively. [ 35 S]GTPγS-binding assay [ 35 S]GTPγS-binding experiments were conducted as described previously [24] , [29] , [32] . In brief, homogenates of membranes of CHO-hM 2 wild-type or CHO-hM 2 W422A cells (40 μg ml −1 ) were incubated with 0.07 nM [ 35 S]GTPγS and maximum agonist-induced [ 35 S]GTPγS incorporation was measured after 1 h. cAMP accumulation assay Agonist-induced rise of intracellular cAMP was captured in CHO-hM 2 cells pretreated with 50 ng ml −1 PTX for 16–24 h as described previously [54] using the HTRF-cAMP dynamic kit (Cisbio, Bagnols-sur-Cèze, France) following the manufacturer's instructions. Fluorescence was quantified on a Mithras LB 940 reader (Berthold Technologies, Bad Wildbad, Germany). ERK1/2 phosphorylation assay Quantification of phosphorylated ERK1/2 levels was performed using the HTRF-Cellul'erk kit (Cisbio). CHO-hM 2 cells were seeded into 96-well plates at a density of 40,000 cells per well and cultured overnight. For PTX pretreatment, cells were dispensed in medium containing 100 ng ml −1 PTX. The next day, cells were washed twice in HBSS buffer supplemented with 20 mM HEPES and starved for 4 h in serum-free medium. After starvation, cells were incubated with agonists diluted in medium for 10 min at 37 °C. Following treatment, agonists were removed and cells were lysed in 50 μl of the supplemented lysis buffer. The plates were incubated for 10 min at room temperature with shaking to lyse the cells and then frozen overnight at −20 °C. Lysates (16 μl) were transferred to a white 384-well plate. Anti-phospho-ERK1/2-d2 (2 μl) and anti-ERK1/2-Eu 3+− Cryptate (2 μl) were added to each well and plates were incubated in the dark for 2 h at room temperature. Time-resolved FRET signals were measured after excitation at 320 nm using the Mithras LB 940 multimode reader (Berthold Technologies). Data analysis was based on the fluorescence ratio emitted by the d2-labelled anti-phospho-ERK1/2 (665 nm) over the light emitted by the Eu 3+ -Cryptate-labelled anti-ERK1/2 (620 nm). Levels of phosphorylated ERK1/2 were normalized to those obtained by 100 μM ACh. BRET assay β-Arrestin2 recruitment assays were performed on HEK293 cells stably expressing GFP2-β-arr2 and transiently coexpressing the human M 2 receptor–Rluc fusion protein and GRK2. For measurement of G-protein subunit rearrangements, COS-7 cells transiently coexpressing the hM 2 receptor, Gα i1 -91Rluc, GFP10-Gγ 2 along with the complementary subunit Gβ 1 were used. Forty-eight hours after transfection, cells were detached and resuspended in HBSS with 20 mM HEPES at a density of 1.06×10 6 cells per ml. Cell suspension (170 μl) was distributed in white 96-well microplates and incubated in the presence of 10 μl buffer or agonist for 2 min (β-arrestin2 recruitment) or 1 min (G-protein activation) before substrate addition. DeepBlueC coelenterazine (Gold Biotechnology, MO, USA; 20 μl per well) was injected by injector 3 to yield a final concentration of 5 μM. To detect BRET, light emission at 400 and 515 nm was measured sequentially using a Mithras LB 940 instrument. The BRET signal (milliBRET ratio) was determined by calculating the ratio of the light emitted by the fluorescence acceptor (515 nm) and the light emitted by Rluc (400 nm). FlAsH labelling and single cell-FRET measurements FlAsH labelling was performed as published previously [43] . In brief, cells were grown to near confluence on glass coverslips. Cells were washed twice with labelling buffer containing 150 mM NaCl, 10 mM HEPES, 2.5 mM KCl, 4 mM CaCl 2 , 2 mM MgCl 2 supplemented with 10 mM glucose (pH 7.3). After incubation with labelling buffer supplemented with 500 nM FlAsH and 12.5 μM 1,2-ethanedithiol (EDT) at 37 °C for 1 h, cells were flushed twice with labelling buffer. To reduce non-specific binding, the cells were again incubated for 10 min with labelling buffer supplemented with 250 μM EDT. Finally, the cells were rinsed twice with labelling buffer. FRET measurements were performed using a Zeiss Axiovert 200 inverted microscope endued with a PLAN-Neofluar oil immersion 100-objective, a dual emission photometric system and a Polychrome IV light source (Till Photonica, Gräfelfing, Germany) as described previously [42] , [44] . Experiments were conducted at room temperature using live HEK293 cells stably expressing the hM 2 receptor FRET-sensor that were maintained in assay buffer. Single cells were excited at 436 nm (dicroic 460 nm) with a frequency of 10 Hz. Emitted light was recorded using 535/30 nm and 480/40 nm emission filters and a DCLP 505 nm beam splitter for FlAsH and CFP, respectively. FRET was observed as the ratio of FlAsH/CFP, which was corrected offline for bleedthrough, direct FlAsH excitation and photobleaching using the 8.0 version of the Origin software as described recently [44] . To investigate changes in FRET on ligand addition, cells were continuously superfused with FRET buffer complemented with various ligands in saturating concentrations as indicated. Superfusion was done using the ALA-VM8 (ALA Scientific Instruments). Calculations and data analysis Quantification of probe-induced DMR signals was based on the signal's peak value between 500 and 1,200 s. All DMR recordings were solvent corrected. All nonlinear regression analyses were performed using Prism 5.01 (GraphPad Software, San Diego, CA). Equilibrium binding data from ACh, iperoxo, iper-6 and iper-8-phth were analysed by a four-parameter logistic function yielding IC 50 values, which were subsequently converted into apparent equilibrium dissociation constants K i using the Cheng-Prusoff correction as described previously [24] . In case of allosteric incomplete displacement of [ 3 H]NMS by iper-6-phth, iper-6-naph and iper-8-naph, curve analysis was based on the allosteric ternary complex model as described elsewhere [24] , [29] . Data obtained from [ 35 S]GPTγS-binding and cAMP accumulation assays were subjected to a two-step analysis. First, data were fitted by a four-parameter logistic function yielding parameter values for a ligand's potency (pEC 50 ) and maximum effect ( E max ). Second, data points were analysed by the operational model of agonism [37] , where E max is the maximal response of the system induced by the maximal effect of a full agonist, K A is the equilibrium dissociation constant of the agonist–receptor complex and reflects affinity, and τ is the 'coupling efficiency', which indicates how efficient agonist binding is transduced into a signalling response and therefore reflects agonist efficacy. For quantification of ligand bias, we used a scale log( τ / K A ) that comprises information about both affinity and efficacy of the respective agonist for activating a signalling pathway [38] . These transduction coefficients were then expressed relative to ACh for each pathway according to To offset the effects of system bias and to display true ligand bias, a 'Log bias' scale is given by Computation of transduction coefficients, ratios thereof and the bias factors included error propagation. Statistical analysis Data are shown as means±s.e.m for n observations. Comparisons of groups were performed using one-way ANOVA or two-way ANOVA with Bonferroni's multiple comparison test. How to cite this article: Bock, A. et al . The allosteric vestibule of a seven transmembrane helical receptor controls G-protein coupling. Nat. Commun. 3:1044 doi: 10.1038/ncomms2028 (2012).